Regulation of tyrosine hydroxylase transcription by hnRNP K and DNA secondary structure Regulation of tyrosine hydroxylase gene ( Th ) transcription is critical for specifying and maintaining the dopaminergic neuronal phenotype. Here we define a molecular regulatory mechanism for Th transcription conserved in tetrapod vertebrates. We show that heterogeneous nuclear ribonucleoprotein (hnRNP) K is a transactivator of Th transcription. It binds to previously unreported and evolutionarily conserved G:C-rich regions in the Th proximal promoter. hnRNP K directly binds to C-rich single-stranded DNA within these conserved regions and also associates with double-stranded sequences when proteins, such as CRE-binding protein, are bound to an adjacent cis -regulatory element. The single DNA strands within the conserved G:C-rich regions adopt either G-quadruplex or i-motif secondary structures. We also show that small molecule-mediated stabilization of these secondary structures represses Th promoter activity. These data suggest that these secondary structures are targets for pharmacological modulation of the dopaminergic phenotype. Dopamine is an essential neurotransmitter for numerous neurological functions that include locomotor behaviours, lactation, light/dark visual adaptation and odour detection. Consistent with its pleiotropic role in the nervous system, dopaminergic dysfunction in humans underlies many debilitating conditions, including Parkinson’s Disease, schizophrenia, depression, drug addiction and attention deficit disorders. These important roles in neurobiology have motivated numerous studies on the molecular mechanisms responsible for development and maintenance of the dopaminergic phenotype. Many studies have concentrated on transcription regulatory mechanisms of tyrosine hydroxylase ( Th ), which encodes the rate-limiting enzyme in catecholamine neurotransmitter biosynthesis. Despite these intense efforts, the transcription factors and molecular mechanisms necessary to generate the complex patterns of Th transcription in the nervous system are only partially understood. Several studies have demonstrated that a cAMP response element (CRE) within the Th proximal promoter region is necessary for mediating transcription in catecholaminergic neurons [1] , [2] , [3] . In humans, single-nucleotide polymorphisms within this site are associated with the neurometabolic disorder Tyrosine Hydroxylase Deficiency [4] . Although necessary, the CRE is not sufficient to establish the complex spatial expression pattern of Th in the brain [5] . NURR1 (NR4A2) is a region-specific transcription factor necessary for Th transcription in midbrain dopaminergic neurons [6] , [7] . The functionality of a putative NURR1-binding site [8] , [9] in the Th proximal promoter is difficult to confirm, however, as it partially overlaps with the TATA box. ETS-domain transcription factors have also been proposed to direct brain region-specific Th expression [10] . We previously showed that the ETS-domain transcription factor ER81 (ETV1) binds the Th promoter in mouse olfactory bulb (OB) dopaminergic neurons, but this molecular mechanism for regulating Th expression is rodent specific [11] . Given the extensive use of rodents to model human dopaminergic systems, a high priority is to identify transcriptional regulatory mechanisms that are conserved between species [12] . To identify functional and evolutionarily conserved transcriptional cis -regulatory elements, we align Th proximal promoter nucleotide sequences from a wide range of vertebrate species. This analysis identifies two novel, conserved G:C-rich regions upstream of the CRE that facilitate Th promoter activity. We show that these regions are bound by heterogeneous nuclear ribonucleoprotein K (hnRNP K) and adopt G-quadruplex and i-motif secondary structures. We also show that small molecule-mediated stabilization of these secondary structures represses Th promoter activity. Together, these findings reveal a novel regulatory mechanism for Th transcription conserved in most vertebrate species and suggest that secondary structures in the Th promoter are novel targets for pharmacological modulation of the dopaminergic phenotype. Conserved functional regions in the Th proximal promoter To identify evolutionarily conserved regions, Th proximal promoter nucleotide sequences from species in five vertebrate orders (mammals, avians, reptiles, amphibians and fish) were aligned. Focusing on the region ~200 base pairs upstream of the transcription start site, the alignment revealed that all tetrapods (mammals, avians, reptiles and amphibians) contain a CRE and TATA box as well as two previously unrecognized G:C-rich regions upstream from the CRE (GC-R1 and GC-R2; Fig. 1a ). The length of these regions varied by species, but both contained several short motifs that were highly conserved. 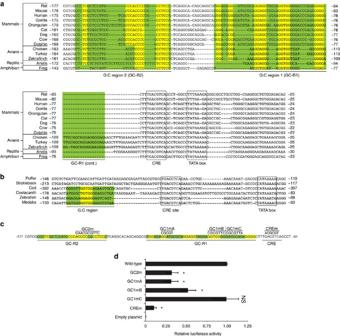Figure 1: Identification of highly conserved and functional G:C-rich regions in the vertebrateThproximal promoters. (a,b) Alignment of vertebrateThproximal promoter nucleotide sequences. (a) TheThproximal promoter of all tetrapod species examined contains two previously unreported G:C-rich regions (GC-R1 and GC-R2; shaded in green). Within these regions, several short nucleotide motifs are highly conserved (shaded in yellow). Both GC-R1 and GC-R2 are upstream of the highly conserved and well-established CRE and TATA box sequences (boxed). (b) In fish, the CRE and TATA box are also conserved, but a single G:C-rich region was found in only a subset of species. Nucleotide positions are numbered relative to the translation start site. (c,d) Functional analysis of G:C-rich regions in theThproximal promoter. (c) Nucleotide sequence of the ratThproximal promoter used for transcription assays. Highly conserved motifs within GC-R1 and GC-R2 are shaded in yellow and mutated positions are shown above the wild-type sequence. The species used for alignment of the proximal promoter sequences were: rat,Rattus norvegicus; mouse,Mus musculus; guinea pig,Cavia porcellus; human,Homo sapiens; Gorilla,Gorilla gorilla; Orangutan,Pongo abelii; cat,Felis catus; dog,Canis familiaris; cow,Bos taurus; dolphin,Tursiops truncatus; chicken,Gallus gallus; turkey,Meleagris gallpavo; zebrafinch,Taeniopygia guttata; anole,Anois carolinensis; frog,Xenopus tropicalis; puffer,Takifugu rubripes; Stickleback,Gasterosteus aculeatus; Zebrafish,Danio rerio; Medaka,Oryzias latipes; Cod;Gadus morhua; Coelancath,Latimeria chalumnae. (d) Luciferase reporter activity in aTh-expressing cell line derived from the mouse olfactory bulb (OB). Mutations overlapping highly conserved nucleotides significantly reduced luciferase reporter activity relative to the wild-type promoter activity (indicated by asterisks;P<0.01 by Student’st-test). By contrast, mutations not overlapping highly conserved nucleotides (that is, GC1mC) did not significantly reduce reporter gene expression (indicated by ‘NS’). Luciferase activities are reported as the mean of three independent transfection experiments with error bars representing the standard error of the mean. Figure 1: Identification of highly conserved and functional G:C-rich regions in the vertebrate Th proximal promoters. ( a , b ) Alignment of vertebrate Th proximal promoter nucleotide sequences. ( a ) The Th proximal promoter of all tetrapod species examined contains two previously unreported G:C-rich regions (GC-R1 and GC-R2; shaded in green). Within these regions, several short nucleotide motifs are highly conserved (shaded in yellow). Both GC-R1 and GC-R2 are upstream of the highly conserved and well-established CRE and TATA box sequences (boxed). ( b ) In fish, the CRE and TATA box are also conserved, but a single G:C-rich region was found in only a subset of species. Nucleotide positions are numbered relative to the translation start site. ( c , d ) Functional analysis of G:C-rich regions in the Th proximal promoter. ( c ) Nucleotide sequence of the rat Th proximal promoter used for transcription assays. Highly conserved motifs within GC-R1 and GC-R2 are shaded in yellow and mutated positions are shown above the wild-type sequence. The species used for alignment of the proximal promoter sequences were: rat, Rattus norvegicus ; mouse, Mus musculus ; guinea pig, Cavia porcellus ; human, Homo sapiens ; Gorilla, Gorilla gorilla ; Orangutan, Pongo abelii ; cat, Felis catus ; dog, Canis familiaris ; cow, Bos taurus ; dolphin, Tursiops truncatus ; chicken, Gallus gallus ; turkey, Meleagris gallpavo ; zebrafinch, Taeniopygia guttata ; anole, Anois carolinensis ; frog, Xenopus tropicalis ; puffer, Takifugu rubripes ; Stickleback, Gasterosteus aculeatus ; Zebrafish, Danio rerio ; Medaka, Oryzias latipes ; Cod; Gadus morhua ; Coelancath, Latimeria chalumnae . ( d ) Luciferase reporter activity in a Th -expressing cell line derived from the mouse olfactory bulb (OB). Mutations overlapping highly conserved nucleotides significantly reduced luciferase reporter activity relative to the wild-type promoter activity (indicated by asterisks; P <0.01 by Student’s t -test). By contrast, mutations not overlapping highly conserved nucleotides (that is, GC1mC) did not significantly reduce reporter gene expression (indicated by ‘NS’). Luciferase activities are reported as the mean of three independent transfection experiments with error bars representing the standard error of the mean. Full size image The alignment of the Th proximal promoter in several fish species revealed similarities to tetrapods. Both a CRE and TATA box motif were identified in all of the fish species examined ( Fig. 1b ). In contrast to tetrapods, however, a G:C-rich region was observed in only a subset of fish species. The G:C-rich region in fish resembled GC-R1 in tetrapods, including the partial conservation of a 5′-GGTGG-3′ sequence. To determine whether the G:C-rich regions modulated Th promoter activity, luciferase transcription assays were performed using the 4.5-kb upstream rat Th promoter in a Th -expressing cell line derived from the mouse OB. The rat 4.5-kb upstream region was used because it is the minimum sequence sufficient for directing Th promoter activity in all catecholaminergic brain regions in transgenic mice [13] . Mutations that overlapped highly conserved residues in both G:C-rich regions substantially reduced reporter gene expression in the OB cell line, but not as much as mutations to the CRE ( Fig. 1c,d ). Mutations within the G:C-rich regions that did not overlap with highly conserved sequences (for example, GC1mC) had little effect on promoter activity. Together, these findings indicate that highly conserved sequences in both G:C-rich regions are functional and important for activating Th transcription. Identification of hnRNP K as a regulator of Th transcription To identify proteins that bind to the G:C-rich regions, pull-down experiments were performed using biotinylated double-stranded oligonucleotides containing either the wild-type or mutated sequences. Initial studies focused on the 5′-GGTGG-3′ sequence in GC-R1 ( Fig. 2a ), as this motif was strongly conserved in vertebrates ( Fig. 1a,b ). The target oligonucleotides were incubated with nuclear lysate from Th -expressing cell lines derived from either the substantia nigra (SN) or the OB. Coomassie-stained gels showed a band that was differentially pulled down in both cell lines ( Fig. 2a ). Mass spectrometry established that this band corresponded to hnRNP K. Transcription assays in human SH-SY5Y cells showed that luciferase activity under the control of the 4.5-kb upstream rat Th promoter was upregulated when hnRNP K was overexpressed ( Fig. 2b ). Human Th promoter activity in SH-SY5Y cells was also upregulated in SH-SY5Y cells ( Supplementary Fig. 1 ). 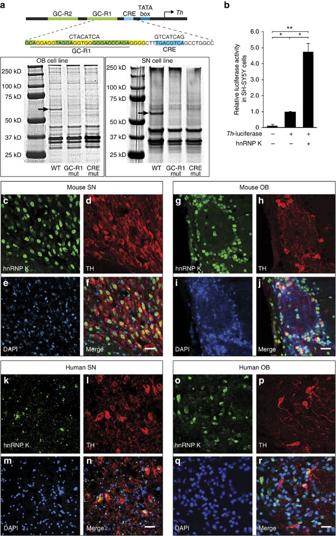Figure 2: hnRNP K interacts with the conserved G:C-rich regions in theThproximal promoter and is co-expressed with THin vivo. (a) Protein pull-down assays with nuclear lysates from mouseTh-expressing cells derived from the mouse olfactory bulb (OB) and substantia nigra (SN). Forward strand of wild-type and mutant oligonucleotide duplexes derived from GC-R1 are shown with mutant positions above the wild-type sequence. Proteins pulled down with either the wild-type or the mutant duplex probes were revealed by coomassie-stained SDS–polyacrylamide gels. Mass spectrometry identified the differentially isolated protein (indicated by arrow) as hnRNP K. (b) Transcription assays in human SH-SY5Y cells showed overexpression of hnRNP K could upregulateThpromoter activity. Luciferase activities are reported as the mean of three independent transfection experiments with error bars representing the standard error of the mean. Pairwise comparisons of luciferase activity levels used the Student’st-test (single asterisk indicatesP<0.01; double asterisk indicatesP<0.001). (c–r) TH and hnRNP K co-expression in mice and humans. In both the SN (c–fandk–n) and OB (g–jando–r), most TH-containing cells co-express hnRNP K. Scale bar, 50 μm. Figure 2: hnRNP K interacts with the conserved G:C-rich regions in the Th proximal promoter and is co-expressed with TH in vivo . ( a ) Protein pull-down assays with nuclear lysates from mouse Th -expressing cells derived from the mouse olfactory bulb (OB) and substantia nigra (SN). Forward strand of wild-type and mutant oligonucleotide duplexes derived from GC-R1 are shown with mutant positions above the wild-type sequence. Proteins pulled down with either the wild-type or the mutant duplex probes were revealed by coomassie-stained SDS–polyacrylamide gels. Mass spectrometry identified the differentially isolated protein (indicated by arrow) as hnRNP K. ( b ) Transcription assays in human SH-SY5Y cells showed overexpression of hnRNP K could upregulate Th promoter activity. Luciferase activities are reported as the mean of three independent transfection experiments with error bars representing the standard error of the mean. Pairwise comparisons of luciferase activity levels used the Student’s t -test (single asterisk indicates P <0.01; double asterisk indicates P <0.001). ( c – r ) TH and hnRNP K co-expression in mice and humans. In both the SN ( c – f and k – n ) and OB ( g – j and o – r ), most TH-containing cells co-express hnRNP K. Scale bar, 50 μm. Full size image Double-label immunofluorescence was used to establish in vivo co-expression of hnRNP K with TH in OB and SN dopaminergic neurons in both mice and humans. This analysis showed that nearly all TH-expressing cells co-expressed hnRNP K in both the mouse SN (217 out of 226 SN TH + cells counted; Fig. 2c–f ) and the OB (131 out of 141 TH + cells counted; Fig. 2g–j ). In tissue obtained from human subjects, most cells with TH also co-expressed hnRNP K in both the SN (159 out of 167 TH + cells counted; Fig. 2k–n ) and OB (134 out of 145 TH + counted; Fig. 2o–r ). In all mouse and human sections examined, there were hnRNP K-expressing cells lacking TH co-expression. Thus, the immunofluorescence data are consistent with a role for hnRNP K in regulating Th transcription, but the presence of hnRNP K + cells lacking TH co-expression indicates that hnRNP K is not sufficient to induce Th transcription. To test whether hnRNP K associated with the Th promoter in a cellular context, we performed chromatin immunoprecipitation (ChIP) assays with SH-SY5Y cells. These studies showed that hnRNP K directly bound the G:C-rich regions of the Th promoter ( Fig. 3a ). Previous studies have shown that hnRNP K preferentially binds C-rich single-stranded DNA sequences [14] . To establish whether hnRNP K binds single DNA strands from the G:C-rich regions in the Th promoter, pull-down assays used single-stranded biotinylated oligonucleotides incubated with nuclear lysate from either OB or SN cell lines. The target oligonucleotide sequences contained either the wild-type G:C-rich region sequences or the mutations overlapping highly conserved positions ( Fig. 3b ). Western blots showed that hnRNP K was preferentially pulled down by the wild-type C-rich strands of both GC-R1 and GC-R2 ( Fig. 3b ; Supplementary Fig. 2 ). 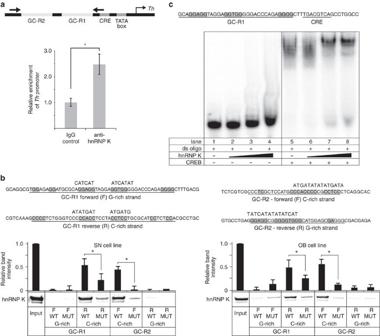Figure 3: hnRNP K binding to theThproximal promoter. (a) Chromatin immunoprecipitation assays with human SH-SY5Y cells indicated that hnRNP K directly binds theThproximal promoter. Three independent ChIP experiments were conducted and the mean relative enrichment of theThproximal promoter is reported with error bars representing the standard error of the mean. Statistical significance was assessed using the two-tailed Student’st-test (asterisk indicatesP<0.01). Arrows show the position on theThpromoter of the primers used in this assay. (b) hnRNP K binds to single-stranded sequences from theThpromoter. Wild-type and mutant oligonucleotides derived from the GC-R1 and GC-R2 are shown with mutated positions above the wild-type sequence. Highly conserved nucleotides within GC-R1 and GC-R2 are shaded. Western blot analyses showed that wild-type C-rich single strands preferentially pulled down hnRNP K from OB and SN cell line nuclear lysates. Band intensities, shown above the blot, are reported as the mean of duplicate pull-down assays with error bars representing the difference between the mean and the individual trials. Compared to the wild-type strands, mutant C-rich strands significantly reduced the interaction with hnRNP K (asterisk indicatesP<0.01 by Student’st-test). (c) The duplex oligonucleotide containing GC-R1 (show on top with highly conserved nucleotides shaded) was not bound by hnRNP K in electromobility shift assays (lanes 1–4). By contrast, hnRNP K did super-shift this target sequence when CREB was present (lanes 5–8). Figure 3: hnRNP K binding to the Th proximal promoter. ( a ) Chromatin immunoprecipitation assays with human SH-SY5Y cells indicated that hnRNP K directly binds the Th proximal promoter. Three independent ChIP experiments were conducted and the mean relative enrichment of the Th proximal promoter is reported with error bars representing the standard error of the mean. Statistical significance was assessed using the two-tailed Student’s t -test (asterisk indicates P <0.01). Arrows show the position on the Th promoter of the primers used in this assay. ( b ) hnRNP K binds to single-stranded sequences from the Th promoter. Wild-type and mutant oligonucleotides derived from the GC-R1 and GC-R2 are shown with mutated positions above the wild-type sequence. Highly conserved nucleotides within GC-R1 and GC-R2 are shaded. Western blot analyses showed that wild-type C-rich single strands preferentially pulled down hnRNP K from OB and SN cell line nuclear lysates. Band intensities, shown above the blot, are reported as the mean of duplicate pull-down assays with error bars representing the difference between the mean and the individual trials. Compared to the wild-type strands, mutant C-rich strands significantly reduced the interaction with hnRNP K (asterisk indicates P <0.01 by Student’s t -test). ( c ) The duplex oligonucleotide containing GC-R1 (show on top with highly conserved nucleotides shaded) was not bound by hnRNP K in electromobility shift assays (lanes 1–4). By contrast, hnRNP K did super-shift this target sequence when CREB was present (lanes 5–8). Full size image On some gene promoters, hnRNP K binds double-stranded DNA sequences [15] , [16] . Electromobility shift assays (EMSAs) with a double-stranded oligonucleotide of the Th promoter, however, did not detect any binding of hnRNP K (lanes 1–4 in Fig. 3c ; Supplementary Fig. 3 ). The inability of hnRNP K to bind this duplex oligonucleotide was unexpected as this was the same duplex used initially to isolate hnRNP K in the protein pull-down experiment ( Fig. 2a ). An important difference between these experiments, however, was that the protein pull-down experiments used nuclear lysate from Th -expressing cell lines, but the EMSA used purified hnRNP K protein. These data suggested that an additional factor in the nuclear lysate enabled hnRNP K to associate with the double-stranded DNA. Given the proximity of the CRE, we tested whether the presence of purified CRE-binding protein (CREB) influenced the binding behaviour of hnRNP K. Additional EMSAs showed that hnRNP K super-shifted CREB/DNA complexes (lanes 5–8 in Fig. 3c ; Supplementary Fig. 3 ). Both the CREB-only and CREB/hnRNP K samples produced multiple shifted bands, suggesting that multiple protein/DNA complexes were present. CREB bound the probe even when the CRE was mutated ( Supplementary Fig. 4 ), which suggested that the multiple protein/DNA complexes in Fig. 3c were generated by CREB recognizing non-canonical, but as yet unidentified, binding sites in the Th promoter. The ability of hnRNP K to super-shift these complexes indicated that proteins bound to the CRE were required to recruit hnRNP K to the duplex Th proximal promoter. To confirm that the CRE was necessary for this recruitment, protein pull-down assays with OB and SN cell line nuclear lysate were performed using a duplex probe derived from GC-R1 with the CRE mutated ( Fig. 2a ). These pull-down experiments differentially isolated a protein that was mass spectrometrically confirmed as hnRNP K, indicating that mutation of the CRE was sufficient to block pull-down of hnRNP K from nuclear lysates of both OB and SN cell lines ( Fig. 2a ). DNA secondary structure in the Th proximal promoter Individual strands of gene promoter regions targeted by hnRNP K can adopt DNA secondary structures that modulate transcription [17] , [18] . C-rich strands can form i-motif structures and the opposing G-rich strands can generate G-quadruplexes [19] . To address whether the Th promoter can also adopt these DNA secondary structures, we examined single-stranded oligonucleotides from GC-R1 and GC-R2 by circular dichroism (CD) spectroscopy. Previous studies have established that i-motifs and G-quadruplexes are stabilized in vitro by low pH (<5) and high K + concentrations (≥100 mM), respectively [20] , [21] . Both wild-type G-rich strands from the Th promoter had similar CD absorption spectra with minima and a maxima that were enhanced in the presence of 100 mM KCl ( Fig. 4a,b ). These spectra also strongly resemble previously reported CD spectra for parallel-stranded G-quadruplexes [22] , [23] , [24] , [25] , [26] . In contrast to the wild-type sequences, mutations to the G-rich sequences from the Th promoter shifted the signal minima and maxima to longer wavelengths and blocked KCl-mediated enhancement of the signal maximum intensity ( Fig. 4a,b ). CD spectra for both wild-type C-rich strands from the Th promoter were consistent with formation of i-motif secondary structures. Lowering the sample pH from 7.6 to 4.6 shifted spectral minimum and maximum to longer wavelengths and strongly enhanced the intensity of the signal maximum ( Fig. 4c,d ). These spectra were nearly identical to previous analyses of i-motif structures by CD spectroscopy [23] , [24] , [27] , [28] . Mutation of the C-rich regions in the Th promoter sequences blocked the pH-induced changes in the CD spectra ( Fig. 4c,d ). Together, the CD spectra strongly indicate that the single-stranded sequences of the Th promoter adopt either G-quadruplex or i-motif secondary structures. 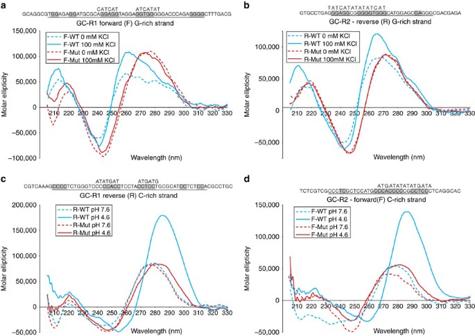Figure 4: Circular dichroism spectra for the single DNA strands from G:C-rich regions in theThproximal promoter. (a,b) Wild-type G-rich single strands (blue lines) show a KCl concentration-dependent enhancement of spectral features. By contrast, spectral features for mutant sequences (red lines) are not KCl concentration dependent. (c,d) Wild-type C-rich single strands (blue lines) show a pH-dependent wavelength shift and enhancement of signal maxima. By contrast, spectral features for the mutant sequences (red lines) are not pH dependent. Oligonucleotide sequences used are displayed above their corresponding spectra with highly conserved motifs within these regions shaded and mutant positions are shown above the wild-type sequence. Figure 4: Circular dichroism spectra for the single DNA strands from G:C-rich regions in the Th proximal promoter. ( a , b ) Wild-type G-rich single strands (blue lines) show a KCl concentration-dependent enhancement of spectral features. By contrast, spectral features for mutant sequences (red lines) are not KCl concentration dependent. ( c , d ) Wild-type C-rich single strands (blue lines) show a pH-dependent wavelength shift and enhancement of signal maxima. By contrast, spectral features for the mutant sequences (red lines) are not pH dependent. Oligonucleotide sequences used are displayed above their corresponding spectra with highly conserved motifs within these regions shaded and mutant positions are shown above the wild-type sequence. Full size image To establish whether DNA secondary structure was present on the Th promoter in vivo , ChIP experiments were performed with the BG4 antibody, which specifically recognizes G-quadruplex structures [29] ( Supplementary Fig. 5 ). In both mouse OB and midbrain tissue, these studies revealed the presence of G-quadruplex structures on the Th promoter in vivo ( Fig. 5a,b ). ChIP experiments also detected G-quadruplexes on the Th promoter in SH-SY5Y cells ( Fig. 5c ). 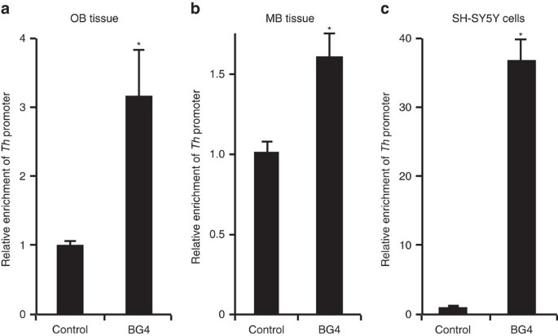Figure 5:In vivoandin vitrodetection of G-quadruplex secondary structures on theThpromoter. (a,b) ChIP experiments with the BG4 antibody detected G-quadruplex secondary structures on theThpromoterin vivoin both the mouse olfactory bulb (OB) and midbrain (MB), respectively. (c) Parallelin vitroChIP studies with human SH-SY5Y cells confirmed the presence of G-quadruplex secondary structures on theThpromoter. For ChIP experiments, three independent immunoprecipitations were performed and the mean relative enrichment of theThproximal promoter is reported with error bars representing the standard error of the mean. Statistical significance was assessed using the two-tailed Student’st-test (asterisks indicateP<0.01). Figure 5: In vivo and in vitro detection of G-quadruplex secondary structures on the Th promoter. ( a , b ) ChIP experiments with the BG4 antibody detected G-quadruplex secondary structures on the Th promoter in vivo in both the mouse olfactory bulb (OB) and midbrain (MB), respectively. ( c ) Parallel in vitro ChIP studies with human SH-SY5Y cells confirmed the presence of G-quadruplex secondary structures on the Th promoter. For ChIP experiments, three independent immunoprecipitations were performed and the mean relative enrichment of the Th proximal promoter is reported with error bars representing the standard error of the mean. Statistical significance was assessed using the two-tailed Student’s t -test (asterisks indicate P <0.01). Full size image The porphyrin compound TMPyP4 ( Fig. 6a ) can stabilize both G-quadruplexes and i-motifs by non-intercalative mechanisms [30] , [31] . By contrast, the structural isomer, TMPyP2 ( Fig. 6a ), is ineffective at stabilizing these DNA secondary structures [32] , [33] , [34] . To establish whether TMPyP4 can stabilize DNA secondary structures formed by the Th promoter DNA, oligonucleotide template strands derived from GC-R1 and GC-R2 were amplified by PCR in the presence of either TMPyP4 or TMPyP2. The presence of TMPyP4, but not TMPyP2, was expected to diminish transcription by stabilizing the DNA secondary structure on the template strands and blocking the DNA polymerase enzyme. These assays showed that increasing TMPyP4 concentrations progressively reduced transcription of the wild-type template strands ( Fig. 6b ). By contrast, the TMPyP2 only weakly reduced or even enhanced transcription product formation rates. Transcription of the mutated template strands also was not significantly impeded by TMPyP4 ( Fig. 6b ). Together, these findings indicate that TMPyP4 can stabilize DNA secondary structures in the Th promoter. 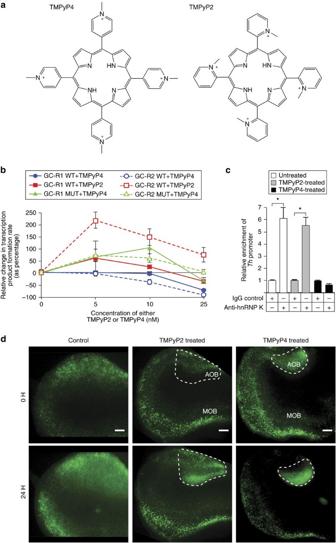Figure 6: Small-molecule manipulation of DNA secondary structure in theThpromoter. (a) The isomeric porphyrin compounds TMPyP4 and TMPyP2 were used as agents to modulate DNA secondary structure stability. (b) Increasing concentrations of TMPyP4, but not TMPyP2, block transcription of template strands derived from the GC-R1 and GC-R2. By contrast, TMPyP4 was not effective at impeding transcription of template strands with mutations to the G:C-rich regions of either GC-R1 or GC-R2 (template oligonucleotides are the same as the sequences used inFig. 4). The data shown are the mean of three independent trials with error bars representing the standard error of the mean. (c) ChIP experiments showed that exposure to TMPyP4, but not TMPyP2, blocked hnRNP K occupancy on theThpromoter in SH-SY5Y cells. For all conditions, three independent ChIP experiments were performed and the mean relative enrichment of theThproximal promoter is reported with error bars representing the standard error of the mean. Statistical significance was assessed using the two-tailed Student’st-test (asterisks indicateP<0.01. (d) Depolarized forebrain organotypic slice cultures show that TMPyP4 and TMPyP2 differentially modulateThpromoter activity in dopaminergic neurons of the main olfactory bulb (MOB). After 24 h of exposure, slices exposed to 100 μM TMPyP4 had substantially lowerTh-GFP expression in MOB dopaminergic neurons. By contrast,Th-GFP expression in these neurons was not diminished in slices treated with either 100 μM TMPyP2 or control conditions. The accessory olfactory bulb (AOB) is distinguished from the MOB by the dotted line. Scale bar, 100 μm. Figure 6: Small-molecule manipulation of DNA secondary structure in the Th promoter. ( a ) The isomeric porphyrin compounds TMPyP4 and TMPyP2 were used as agents to modulate DNA secondary structure stability. ( b ) Increasing concentrations of TMPyP4, but not TMPyP2, block transcription of template strands derived from the GC-R1 and GC-R2. By contrast, TMPyP4 was not effective at impeding transcription of template strands with mutations to the G:C-rich regions of either GC-R1 or GC-R2 (template oligonucleotides are the same as the sequences used in Fig. 4 ). The data shown are the mean of three independent trials with error bars representing the standard error of the mean. ( c ) ChIP experiments showed that exposure to TMPyP4, but not TMPyP2, blocked hnRNP K occupancy on the Th promoter in SH-SY5Y cells. For all conditions, three independent ChIP experiments were performed and the mean relative enrichment of the Th proximal promoter is reported with error bars representing the standard error of the mean. Statistical significance was assessed using the two-tailed Student’s t -test (asterisks indicate P <0.01. ( d ) Depolarized forebrain organotypic slice cultures show that TMPyP4 and TMPyP2 differentially modulate Th promoter activity in dopaminergic neurons of the main olfactory bulb (MOB). After 24 h of exposure, slices exposed to 100 μM TMPyP4 had substantially lower Th -GFP expression in MOB dopaminergic neurons. By contrast, Th -GFP expression in these neurons was not diminished in slices treated with either 100 μM TMPyP2 or control conditions. The accessory olfactory bulb (AOB) is distinguished from the MOB by the dotted line. Scale bar, 100 μm. Full size image Stabilization of DNA secondary structure on the Th promoter by TMPyP4 would be expected to preclude proteins, such as hnRNP K, from binding the single-stranded promoter DNA. Consistent with this mechanism, ChIP experiments conducted with SH-SY5Y cells showed reduced hnRNP K occupancy on the Th promoter when the cells were treated with TMPyP4 ( Fig. 6c ). To address whether small molecules, such as TMPyP4, can modulate Th transcription levels in a cellular context, we analysed the effect of these compounds in depolarized forebrain organotypic slice cultures from a transgenic Th -GFP mouse strain expressing green fluorescent protein (GFP) under the control of the 9-kb upstream region of the Th promoter [35] . Compared with either TMPyP2-treated or control sections, GFP expression was strongly attenuated in the main OB dopaminergic neurons of TMPyP4-treated sections ( Fig. 6d ). These findings show that, when provided access to the brain, pharmacological agents that stabilize G-quadruplex and i-motif DNA secondary structures, such as TMPyP4, can modulate Th expression levels. Interestingly, TMPyP4 did not substantially disrupt GFP expression in the accessory OB ( Fig. 6d ). The GFP-expressing cells in the accessory OB are unlikely catecholaminergic neurons as they do not express TH protein ( Supplementary Fig. 6 ), which suggests that Th is differentially regulated in non-catecholaminergic cells. This study identified a novel transcription regulatory mechanism on the Th promoter mediated by hnRNP K and DNA secondary structure. These studies showed that hnRNP K is a transactivator of Th transcription that directly binds C-rich single-stranded DNA sequences within conserved G:C-rich regions of the Th promoter. hnRNP K is an established transactivator targeting C-rich single-stranded DNA sequences of several oncogenes [15] , [16] , [18] , [36] . To our knowledge, however, this is the first study showing that hnRNP K also targets neurotransmitter biosynthesis genes. These studies also found that hnRNP K can associate with duplex DNA sequences from the Th promoter, but only when proteins, such as CREB, are bound to the CRE. Previous reports also demonstrated hnRNP K binding to DNA duplexes [15] , [16] , but these studies used either whole or partially purified nuclear extracts and it is unclear whether additional proteins within the extracts assisted hnRNP K binding to the target duplex sequences. By contrast, the EMSAs reported here used only purified stocks of hnRNP K and CREB proteins. Thus, the DNA-binding synergy was not mediated by third party proteins bridging hnRNP K and CREB. These findings suggest an interaction between hnRNP K and CREB, but protein immunoprecipitation assays have failed to detect any evidence of a specific physical interaction between these two proteins ( Supplementary Fig. 7 ). The inability to co-immunoprecipitate the proteins, however, may be because the interaction between these proteins masks the epitopes necessary for such experiments to detect them. Alternatively, deformations from canonical B-form duplex DNA structure induced by basic-leucine-zipper (bZIP) DNA-binding domain proteins, such as CREB [37] , [38] , may be specifically recognized by hnRNP K and/or integral to the stability of hnRNP K/dsDNA complexes. Together, hnRNP K and bZIP proteins likely co-regulate Th transcription in most dopaminergic neurons. The co-expression of hnRNP K with Th promoter in both the OB and SN suggests that its regulatory function is not region specific. Previous studies have established that the CRE in the Th proximal promoter is required for Th transcription in all catecholaminergic neurons [1] , [2] , [3] , [39] , [40] . The specific bZIP protein complexes bound to the CRE, however, may be region specific. We showed CREB bound the Th promoter in this study, but other bZIP proteins, including Fos-B and Jun-D, can also bind the CRE [41] . Both hnRNP K and bZIP proteins also contact the general transcription protein machinery. hnRNP K physically interacts with the TBP subunit of TFIID, whereas bZIP proteins recruit co-activators, such as CBP/p300, that interact with several subunits of the RNA polymerase II protein complex [42] , [43] , [44] . Thus, both bZIP and hnRNP K proteins are important regulators of the dopaminergic neuronal phenotype through their interactions on the Th promoter. This study also revealed that individual strands from the conserved G:C-rich regions in the Th promoter adopt either G-quadruplex or i-motif secondary structures. This mirrors previous studies showing that these types of DNA secondary structures form on G:C-rich regions of oncogene promoters also targeted by hnRNP K [17] , [18] . The conserved function of hnRNP K and DNA secondary structure on both Th and oncogene promoters leads us to propose that the Th proximal promoter regulates transcription by a mechanism similar to what has been suggested for the c-myc oncogene [17] ( Fig. 7 ). On the Th promoter, the recruitment of bZIP proteins and their co-activators to the CRE facilitates assembly of the RNA polymerase transcription machinery. Melting of core promoter duplex DNA by the RNA polymerase complex generates negative supercoiling upstream of the complex that can promote separation of duplex DNA strands. The resulting single strands can adopt secondary structures, such as G-quadruplexes and i-motifs, which help dissipate the torsional stress [45] . These DNA secondary structures, especially G-quadruplexes, are associated with transcriptional repression through mechanisms that are not established, but may include disruption of transcription elongation, blocking the binding of transcription activator proteins or recruitment of transcription repressor proteins [37] , [38] . By contrast, binding of the single DNA strands by proteins such as hnRNP K prevents secondary structure formation and promotes gene transcription by contacting general transcription factors, such as TBP [42] , [43] . The loss of hnRNP K function in vivo would be expected to reduce Th transcription levels because of both the lost interaction with TBP and the increased rate of secondary structure formation. The lack of hnRNP K knock-out mouse strains, however, has precluded direct testing of this prediction. Alternative strategies to knock down hnRNP K by RNA interference in several neural cell lines using either transfection or lentiviral transduction have been impeded by hnRNP K’s regulation of proliferation and survival genes [46] . 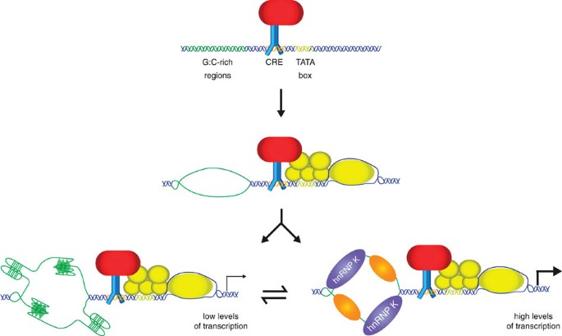Figure 7: Proposed regulatory mechanism for hnRNP K and DNA secondary structure on theThproximal promoter. Recruitment of bZIP proteins (in blue) and associated co-activator proteins (in red) to the CRE facilitates assembly of the RNA polymerase transcription protein complex (in yellow; top panel). Melting of the duplex core promoter DNA by the transcription protein complex generates torsional stress that drives the separation of the duplex DNA in the G:C-rich regions (in green; middle panel). These single DNA strands from the G:C-rich regions either adopt secondary structures, such as G-quadruplexes or i-motifs (bottom left panel), or are bound by proteins such as hnRNP K (bottom right panel).Thtranscription is diminished when secondary structures are formed, whereas stabilization of the unfolded single strands in the G:C-rich regions enhances transcription. Figure 7: Proposed regulatory mechanism for hnRNP K and DNA secondary structure on the Th proximal promoter. Recruitment of bZIP proteins (in blue) and associated co-activator proteins (in red) to the CRE facilitates assembly of the RNA polymerase transcription protein complex (in yellow; top panel). Melting of the duplex core promoter DNA by the transcription protein complex generates torsional stress that drives the separation of the duplex DNA in the G:C-rich regions (in green; middle panel). These single DNA strands from the G:C-rich regions either adopt secondary structures, such as G-quadruplexes or i-motifs (bottom left panel), or are bound by proteins such as hnRNP K (bottom right panel). Th transcription is diminished when secondary structures are formed, whereas stabilization of the unfolded single strands in the G:C-rich regions enhances transcription. Full size image On the c-myc promoter, the CNBP and hnRNP K proteins stabilize the G-rich and C-rich single strands, respectively [17] . In both the OB and SN, we show that the C-rich sequences are also targeted by hnRNP K. Given the broad expression pattern of hnRNP K in the nervous system, we expect that the role of hnRNP K in regulating Th expression is general and not region specific. The factors bound to the G-rich sequences on the Th promoter have not been established, but in a subset of dopaminergic neurons in both the OB and SN, the G-rich regions may be stabilized by hnRNP A1 ( Supplementary Figs 8–10 ). Further testing will establish whether secondary structures on the Th promoter are destabilized by proteins, such as NM23-H2, as they are on the c-myc promoter [17] , [45] . The ability of TMPyP4 to repress Th expression suggests that DNA secondary structures on the Th promoter are novel pharmacological targets for small molecules. This method of repressing Th transcription could assist stem cell engineering protocols to produce non-catecholaminergic neuronal phenotypes. Current pharmacological efforts are concentrated on developing compounds that stabilize the G-quadruplexes in order to repress oncogene expression and telomerase activity [47] , but development of agents that destabilize these structures on Th promoter may benefit therapeutic strategies to treat dopamine-related disorders, such as TH deficiency and Parkinson’s Disease. Recent studies indicate that G-quadruplexes are pervasive throughout the human genome and present in many gene promoter regions [48] , which raises the possibility that pharmacological manipulation of DNA secondary structure may benefit additional neurological conditions. The conservation of the G:C-rich regions, CRE and TATA box in most vertebrate species indicates that the proteins bound to these conserved regions and DNA secondary structure are together part of an evolutionarily ancient mechanism regulating Th transcription. An important future direction is to establish how this mechanism interacts with other transcription factors previously identified as regulators of Th transcription. Understanding how NURR1 integrates with this mechanism is of particular interest. NURR1 is necessary for the development of midbrain dopaminergic neurons and activates the expression of several genes necessary for this phenotype, including Th and c-Ret [6] , [7] , [49] , [50] . Interestingly, the c-Ret promoter can also adopt G-quadruplex and i-motif secondary structures [23] and suggests that similar mechanisms identified here for Th may be also functional on other genes necessary for specifying the dopaminergic phenotype. Genomic sequence alignment All Th proximal promoter genomic sequences were obtained from Ensembl.org ( http://ensembl.org ). For all species, 500 bp sequences upstream from the translation start site were simultaneously aligned and visualized using Multi-LAGAN and mVISTA web-based services ( http://genome.lbl.gov/vista/mvista/submit.shtml ) [51] , [52] . The Ensembl.org gene identifiers for Th in each species: rat, Rattus norvegicus ENSRNOG00000020410; mouse, Mus musculus ENSMUSG00000000214; guinea pig, Cavia porcellus ENSCPOG00000012591; human, Homo sapiens ENSG00000180176; Gorilla, Gorilla gorilla ENSGGOG00000003978; Orangutan, Pongo abelii ENSPPYG00000002924; cat, Felis catus ENSFCAG00000006939; dog, Canis familiaris ENSCAFG00000010099; cow, Bos taurus ENSBTAG00000026768; dolphin, Tursiops truncatus ENSTTRG00000015465; chicken, Gallus gallus ENSGALG00000006551; turkey, Meleagris gallpavo ENSMGAG00000007908; zebrafinch, Taeniopygia guttata ENSTGUG00000009295; anole, Anois carolinensis ENSACAG00000009753; frog, Xenopus tropicalis ENSXETG00000014030; puffer, Takifugu rubripes ENSTRUG00000009267; Stickleback, Gasterosteus aculeatus ENSGACG00000011104; Zebrafish, Danio rerio ENSDARG00000030621; Medaka, Oryzias latipes ENSORLG00000018964; Cod; Gadus morhua ENSGMOG00000017881; Coelancath, Latimeria chalumnae ENSLACG00000006317. Cell culture Generation of the SN-derived Th -expressing cell line (SN4741) has been previously described [53] . Briefly, this clonal cell line was established from mesencephalic tissue dissected from embryonic day 13.5 transgenic mice expressing the SV40 large T-antigen under the control of the rat 9 kb Th upstream region. The OB Th -expressing cell line (OB4671) is also a clonal line derived from this transgenic mouse strain, but it was generated using OB tissue dissected from postnatal day 2 animals. Both OB and SN cell lines were maintained at 33 °C with 95% air and 5% CO 2 on primaria-coated culture dishes in DMEM cell culture medium supplemented with 10% fetal bovine serum and 1% penicillin/streptomycin. The human SH-SY5Y neuroblastoma cell line was maintained at 37 °C with 95% air and 5% CO 2 in DMEM/F12 media supplemented with 10% fetal bovine serum and 1% penicillin/streptomycin. Luciferase transcription assays Transcription assays in the OB cell line were conducted with stably transfected cells. For each line, 2.5 × 10 6 cells in 60-mm Primaria-coated culture dishes were transfected using Fugene HD transfection reagent (Roche) with 2 μg of pGL4.20 firefly luciferase reporter plasmid (Promega). The firefly luciferase was under the control of the rat 4.5 kb Th upstream region containing either the wild-type or the mutated G:C-rich regions. The pGL4.20 plasmid also constitutively expressed a puromycin resistance gene to enable selection of transfected cells. Forty-eight hours after transfection, culture media were supplemented with 25 μg ml −1 puromycin to select transfected cells. The puromycin concentration was reduced to 8.3 μg ml −1 after one subculture and this reduced level was used to maintain the lines. To measure luciferase activity in stably transfected cell lines, cultures were dissociated with trypsin, washed and resuspended in 1 ml of PBS. The density (OD) of the isolated cells was measured at a wavelength of 600 nm. Cells were then pelleted and treated with reporter lysis buffer (Promega). Using a firefly luciferase assay kit (Promega), luminescence was measured with LMaxII luminometer (Molecular Devices). Luminescence readings were normalized to the respective cell densities. Luciferase activity was reported as the mean of three independent transfection experiments with error bars representing the standard error of the mean. Significant changes in activity were assessed either by two-tailed Student’s t -test or by analysis of variance with appropriate post-hoc tests. Transcription assays with SH-SY5Y cells overexpressing hnRNP K were conducted using transient transfections with Lipofectamine LTX transfection reagent (Life Technologies). These experiments used the pGL4.20 plasmid (Promega) with a firefly luciferase reporter gene under the control of the wild-type rat 4.5 kb upstream region and a pGFP-hnRNP K expression plasmid (a generous gift from Dr Rama Natarajan, Beckman Research Institute). To control for variations in transfection efficiency, cells were also transfected with pRL-CMV (Promega), which constitutively expressed Renilla luciferase. Cells were transfected according to the manufacturer’s protocol and maintained for 48 h before both firefly and Renilla luciferase activities were measured using the Dual-Glo Luciferase Assay System (Promega). Luminescence was measured with LMaxII luminometer (Molecular Devices). Luciferase activity was reported as the mean of three independent transfection experiments with error bars representing the standard error of the mean. Significant changes in activity were assessed either by two-tailed Student’s t -test or by analysis of variance with appropriate post-hoc tests. Protein pull-down and mass spectrometry analysis Protein pull-down assays using biotinylated DNA oligonucleotides were based on a previous study with minor modifications [54] . Th -expressing OB and SN cell lines were grown to a density of 10 5 cells per ml on 100 mm primaria-coated culture dishes before being collected and lysed in RIPA buffer supplemented with protease inhibitors. Cellular debris was cleared from the lysate using centrifugation and protein content was estimated by a Bradford Assay (Bio-Rad). Immobilized DNA oligonucleotides were prepared by incubating 20 μg of annealed duplex oligonucleotides with 100 μg of streptavidin-coated Dynabeads (Life Technologies) in 400 μl of buffer (10 mM Tris, pH 7.5, 1 mM EDTA, 1 M NaCl, 0.003% NP40) for 1 h at room temperature with constant rotation. To minimize nonspecific interactions, the immobilized oligonucleotides were incubated for 30 min at room temperature with 2.5 mg ml −1 of BSA in 10 mM HEPES, pH 7.6, 100 mM potassium glutamate, 2.5 mM dithiothreitol (DTT), 10 mM magnesium acetate, 5 mM EGTA, 3.5% glycerol with 0.003% NP40 and 5 mg ml −1 of polyvinylpyrrolidone. Cell lysate containing 100 μg of protein was then incubated with immobilized oligonucleotides for 4 h at 4 °C with constant rotation in 400 μl of 10 mM HEPES, pH 7.6, 100 mM potassium glutamate, 80 mM KCl, 2.5 mM DTT, 10 mM magnesium acetate, 5 mM EGTA, 3.5% glycerol with 0.001% NP40 and 1 μg of nonspecific carrier DNA. After 4 h, the immobilized protein/DNA oligo complexes were washed three times with 300 μl of 10 mM HEPES, pH 7.6, 100 mM potassium glutamate, 2.5 mM DTT, 10 mM magnesium acetate, 5 mM EGTA, 3.5% glycerol, 0.5 mg ml −1 BSA and 0.05% NP40. Proteins bound to the immobilized DNA were eluted in 50 μl of SDS–polyacrylamide gel electrophoresis sample buffer and resolved by electrophoresis on a NuPAGE 4–12% gradient Bis–Tris gel (Life Technologies). The gel was stained with Coomassie Brilliant Blue R-250 (Boston Bioproducts) overnight and destained with a solution of 30% methanol, 7% acetic acid and 63% water. Gels were digitally scanned for image archiving and bands of interest were identified for further analysis. Gels were sent to the Cornell University Life Sciences core mass spectrometry and proteomics facility. This core facility excised the bands of interest, performed in-gel proteolytic digestion and protein fragment extraction. Protein fragments were analysed by matrix-assisted laser desorption/ionization–time of flight mass spectrometry and compared with proteomic databases using Mascot 2.2 software to identify the parent protein. The duplex oligonucleotides used for protein pull-down assays corresponded to rat Th genomic positions −115 to −64 (relative to the start of translation). The wild-type forward strand (biotinylated): 5′-GCAGGAGGTAGGAGGTGGGGGACCCAGAGGGGCTTTGACGTCAGCCTGGCC-3′. The wild-type reverse strand: 5′-GGCCAGGCTGACGTCAAAGCCCCTCTGGGTCCCCCACCTCCTACCTCCTGC-3′. The GC-R1 mutant forward strand (biotinylated; mutated positions underlined): 5′-GCAGGAGGTAGG CTACATCA GACCCAGAGGGGCTTTGACGTCAGCCTGGCC-3′. The GC-R1 mutant reverse strand (mutated positions underlined): 5′-GGCCAGGCTGACGTCAAAGCCCCTCTGGGTC TGATGTAG CCTACCTCCTGC-3′. The CRE mutant forward strand (biotinylated; mutated positions underlined): 5′-GCAGGAGGTAGGAGGTGGGGGACCCAGAGGGGCTT GTCATCAG GCCTGGCC-3′. The CRE mutant reverse strand (mutated positions underlined): 5′-GGCCAGGC CTGATGAC AAGCCCCTCTGGGTCCCCCACCTCCTACCTCCTGC-3′. hnRNP K pull-down assays one microgram of single-stranded biotinylated DNA oligonucleotide was incubated with 5 μg of streptavidin-coated Dynabeads (Life Technologies) in 300 μl of streptavidin-biotin-binding buffer (10 mM Tris, pH 7.5, 1 mM EDTA, 1 M NaCl, 0.003% NP40) at room temperature for 20 min. To minimize nonspecific interactions, the oligo-bead complexes were incubated for 30 min with a blocking buffer (2.5 mg ml −1 BSA in 10 mM HEPES, pH 7.6, 100 mM potassium glutamate, 2.5 mM DTT, 10 mM magnesium acetate, 5 mM EGTA, 3.5% glycerol with 0.003% NP40 and 5 mg ml −1 polyvinylpyrrolidone). Th -expressing OB and SN cell lines were grown in 10 mm dishes and collected at 80% confluence. A total of 3 × 10 7 cells were lysed and the nuclei were extracted with NE-PER nuclear and cytoplasmic extraction reagents (Thermo Scientific). Immobilized oligonucleotides were incubated with 100 μg of nuclear extract for 1 h at 4 °C with constant rotation in 400 μl of protein-binding buffer (10 mM HEPES, pH 7.6, 100 mM potassium glutamate, 80 mM KCl, 2.5 mM DTT, 10 mM magnesium acetate, 5 mM EGTA, 3.5% glycerol with 0.001% NP40 and 1 μg of nonspecific carrier DNA). Protein–DNA complexes were then washed three times (10 mM HEPES, pH 7.6, 100 mM potassium glutamate, 2.5 mM DTT, 10 mM magnesium acetate, 5 mM EGTA, 3.5% glycerol, 0.5 mg ml −1 BSA and 0.05% NP40). Proteins bound to the oligonucelotides were then eluted with 10 μl of denaturing Laemmli sample loading buffer at 37 °C for 15 min. hnRNP K protein in the supernatant was visualized by western blot with a rabbit anti-hnRNP K antibody (Abcam) at 1:2,000 dilution using an Odyssey imaging system (Li-Cor Biosciences). Band intensities were quantified using ImageJ software (National Institutes of Health) and are reported as the mean of duplicate pull-down assays with error bars representing the difference between the mean and the individual trials. The oligonucleotide sequences used in the experiments were: wild-type GC-R1 forward strand, 5′-GCAGGCGTGGAGAGGATGCGCAGGAGGTAGGAGGTGGGGGACCCAGAGGGGCTTTGACG-3′; mutant GC-R1 forward strand (mutated positions underlined), 5′-GCAGGCGTGGAGAGGATGCGC CATCATTAGGAATCATAT GACCCAGAGGGGCTTTGACG-3′; wild-type GC-R1 reverse strand, 5′-CGTCAAAGCCCCTCTGGGTCCCCCACCTCCTACCTCCTGCGCATCCTCTCCACGCCTGC-3′; mutant GC-R1 reverse strand (mutated positions underlined), 5′- CGTCAAAGCCCCTCTGGGTC ATATGATTCCTAATGATG GCGCATCCTCTCCACGCCTGC-3′; wild-type GC-R2 forward strand, 5′- TCTCGTCGCCCTCGCTCCATGCCCACCCCCGCCTCCCTCAGGCAC-3′; mutant GC-R2 forward strand (mutated positions underlined), 5′-TCTCGTCGCCCTCGCTCCATGC ATGATATATATGATA TCAGGCAC-3′; wild-type GC-R2 reverse strand, 5′-GTGCCTGAGGGAGGCGGGGGTGGGCATGGAGCGAGGGCGACGAGA-3′; mutant GC-R2 reverse strand (mutated positions underlined), 5′-GTGCCTGA TATCATATATATCAT GCATGGAGCGAGGGCGACGAGA-3′. Electrophoretic mobility shift assay Both duplex and single-stranded oligonucleotides were end-labelled with γ-P 32 dATP using T4 polynucleotide kinase (New England Biolabs) and unincorporated nucleotides were removed using Bio-30 spin columns (Bio-Rad). All protein-DNA binding reactions were conducted in 20 μl solutions containing 5 mM HEPES (pH 7.9), 25 mM KCl, 0.05 mM EDTA, 0.125 mM phenylmethysulfonyl fluoride, 1 mg ml −1 of nonspecific herring sperm carrier DNA, 0.0 l% NP40 and 2 μl of radiolabelled DNA probe. Binding reactions either used purified protein stocks of hnRNP K (Abcam) or CREB (generous gift from Dr Jennifer K. Nyborg, Colorado State University). Binding reactions were carried out at 4 °C for 1 h before being resolved on either 3 or 5% 29:1 acrylamide/ bis -acrylamide gels with 1/4 × TBE buffer at 215 V for 2 h. Gels were dried and then imaged using a BAS2500 phosphoimager (GE Healthcare). The duplex oligonucleotides used for the EMSAs were the same as the wild-type sequences used for the protein pull-down assays and mass spectrometry analysis (see above). Immunohistology and antibodies Immunohistological analyses in mice used tissue from adult C57BL6 mice that were anaesthetized with an overdose of pentobarbital (100 mg kg −1 ) and perfused transcardially with phosphate-buffered 4% formaldehyde. Brains were removed and post-fixed for 4 h before being cryo-protected in 30% sucrose and cut in 30 μm sagittal sections. Human OB tissue was provided by the Harvard Brain Tissue Resource Center (HBTRC) and the human SN tissue was provided by the New York Brain Bank (NYBB)/Taub Institute for Research on Alzheimer's Disease and the Aging Brain. Tissue was provided from individuals without evidence of neurodegeneration, but the donor selection process was conducted exclusively by the HBTRC and NYBB. As such, all consent forms and patient information are maintained under protocols established by the HBTRC and NYBB, which are sanctioned by Institutional Review Boards approved by the National Institutes of Health. All human tissue samples were obtained postmortem and formalin-fixed before being cryo-protected in 30% sucrose and cut into 30 μm sagittal sections. Antigen retrieval was performed on all human tissue sections by immersing sections in 100 mM Tris (pH 9) with 10 mM glycine overnight at 75 °C, then allowing sections to cool to room temperature before being washed with PBS. For both mouse and human tissue, sections were blocked with 1% BSA in PBS for 1 h before overnight incubation with primary antibody. The rabbit anti-hnRNP K (Abcam) primary antibody was used at a 1:500 dilution. The mouse TH primary antibody (Immunostar) was used at 1:1,000. All primary antibodies were visualized with Alexa-Fluor secondary antibodies (Life Technologies) at a 1:400 dilution. Sections were imaged on either a Nikon 80i Eclipse fluorescence microscope or a Zeiss Meta 500 scanning laser confocal microscope. ChIP assays ChIP experiments to detect hnRNP K occupancy on the Th promoter used SH-SY5Y cells grown in 10 mm culture dishes to 90% confluence before being washed with PBS, and then cross-linked with 1% formaldehyde in PBS at room temperature for 9 min. For ChIP experiments probing the effect of either TMPyP4 or TMPyP2 exposure on hnRNP K occupancy, cells were treated with 100 mM TMPyP4 or TMPyP2 for 24 h before being washed and cross-linked with formaldehyde. Fixation was terminated by addition of 125 mM glycine and the cells were washed twice with PBS before being collected with a sterile cell scraper. Cells were pelleted at 800 g centrifugation at 4 °C for 5 min. The pellet was washed with PBS before lysing the cells with SDS Lysis Buffer (Millipore) and the chromatin was sheared with a Bioruptor (Diagenode). Immunoprecipitation of cross-linked protein/DNA complexes were performed using the Magna ChIP Protein-A/G kit (Millipore) following the manufacturer’s instructions. Immunoprecipitation reactions used 4 μg of either rabbit anti-hnRNP K antibody (Abcam) or normal rabbit IgG (Santa Cruz) and reverse cross-linking was done overnight in the presence of Proteinase K at 62 °C with shaking. Immunoprecipitated Th promoter genomic DNA fragments were amplified and quantified using a 7,500 Fast Real-time PCR System (Applied Biosystems) and SYBR Green PCR master mix (Applied Biosystems). Primer sequences used for amplifying the G:C-rich regions of the Th proximal promoter were 5′-CTGCGCCTCCCTCCTTCCTCAC-3′ and 5′-GAGCTGACGTCAAAGCCCCCTCTG-3′. For all hnRNP K ChIP experiments, three independent experiments were conducted and the mean relative enrichment of the Th proximal promoter is reported with error bars representing the standard error of the mean. Statistical significance was assessed using the two-tailed Student’s t -test. ChIP experiments to detect G-quadruplex secondary structures on the Th promoter used a His/FLAG-tagged BG4 single chain antibody [29] . An expression plasmid for this antibody was generously provided by Dr Shankar Balasubramnian (Cambridge, UK). Control experiments used His-tagged thioredoxin expressed from a pET-32a expression plasmid (Novagen/EMD Millipore). Both His-tagged BG4 and Thioredoxin proteins were generated with BL21(DE3) E. coli cells. An overnight growth was used to inoculate 300 ml of LB media to an OD 600 of 0.1, which was then cultured at 37 °C with shaking. When the OD 600 reached 0.6, protein expression was induced with 1 mM IPTG (Calbiochem). Six hours after induction, cells were spun down and the pellet was washed with PBS before being resuspended in 1.6 ml of equilibration buffer (PBS, with 10 mM imidazole, pH 7.4, and 1 mM phenylmethyl sulphonyl fluoride). The resuspended cells were placed on ice, lysed by sonication and cellular debris was removed by centrifugation. Lysate with equivalent loads of either BG4 or Thioredoxin was incubated on HisPur Ni-NTA resin (Thermo Scientific) at 4 °C for 2 h, after which sheared chromatin from either SH-SY5Y cells, adult male and female Th -GFP mouse tissue from either the OB or the midbrain tissue, was added and incubated at 4 °C overnight. The BG4/Thioredoxin-bound resin was washed three times with 1 × PBS containing 25 mM imidazole, and eluted in PBS with 1 mM EDTA and 25 mM imidazole. Samples were reverse cross-linked overnight at 62 °C on a shaker with 1 μg of Proteinase K. DNA was purified using MinElute PCR purification columns (Qiagen) and Th promoter genomic DNA fragments were amplified and quantified using a 7,500 Fast Real-time PCR System (Applied Biosystems) and SYBR Green PCR master mix (Applied Biosystems). Data are presented as the mean from three independent ChIP experiments with error bars representing the standard error of the mean. Statistical significance was assessed using two-tailed Student’s t -tests. Primer sequences used to amplify the G:C-rich regions of the human Th proximal promoter (from SH-SY5Y cells) were: 5′-CTGCGCCTCCCTCCTTCCTCAC-3′ and 5′-GAGCTGACGTCAAAGCCCCCTCTG-3′. Primer sequences used to amplify the G:C-rich regions of the mouse Th proximal promoter (from OB and midbrain tissue) were: 5′-GTCGCCCTCGCTCTGTGCCCA-3′ and 5′-GGCTGACGTCAAAGCCCCTCTGG-3′. CD experiments CD experiments were performed with an Aviv 414 CD spectrophotomer. All spectra were collected with a wavelength range from 200 to 330 nm, 1 nm step widths and 1 s dwell times. Displayed spectra for each sample are an average of three scans. DNA oligonucleotide sequences used for these studies were identical to those used for the hnRNP K pull-down assays (see above) and all were used at concentrations of 5 μM. For both wild-type and mutant G-rich sequences from GC-R1 and GC-R2, samples were in Tris buffer at pH 7.4 with either 0 or 100 mM KCl. For both wild-type and mutant C-rich sequences from GC-R1 and GC-R2, samples were in sodium citrate/phosphate buffer at either pH 7.6 or 4.6. PCR interference assays with TMPyP4 and TMPyP2 All PCR reactions were performed on a 7,500 Fast Real-time PCR System (Applied Biosystems) using SYBR Green PCR master mix (Applied Biosystems) with 0, 5, 10 or 25 nM of either TMPyP4 (Sigma-Aldrich) or TMPyP2 (Frontier Scientific). The data shown are the mean of three independent trials with error bars representing the standard error of the mean. Both wild-type and mutant oligonucleotide template strands were the same as those used in the hnRNP K pull-down experiments (see above). Primer annealing to the GC-R1 wild-type and mutant forward strand: 5′-AGTCAGTCCGTCAAAG-3′. Primer annealing to the GC-R1 wild-type and mutant reverse strand: 5′-AGTCAGTCGCAGGCGT-3′. Primer annealing to the GC-R2 wild-type and mutant forward strand: 5′-AGTCAGTCGTGCCTGA-3′. Primer annealing to the GC-R2 wild-type and mutant reverse strand: 5′-AGTCAGTCTCTCGTCG-3′. Animals Transgenic Th -GFP mice were obtained from Dr Kazuto Kobayashi [35] . All mice were housed in humidity-controlled cages at 22 °C under a 12:12 h light/dark cycle and provided with food and water ad libitum . All procedures were carried out under protocols approved by the Weill Cornell Medical College Institutional Animal Care and Use Committee and conformed to NIH guidelines. Organotypic slice cultures Whole brains from male and female Th -GFP mouse pups ranging in age from postnatal day 3 or 4 were dissected and placed into Petri dishes containing ice-cold dissection medium (Leibovitz’s L-15 media, pH 7.4; Life Technologies). Brains were transected mid-sagittally and each hemisphere was placed with the medial face down into a plastic tissue embedding mold (Polysciences) and embedded in warm (37 °C) 4% low-melting-point agarose (Sigma) in L-15 medium, then rapidly cooled on ice and cut into 200 μm sagittal slices with a vibratome (Model 1000; Ted Pella Inc.). Slices were cultured in depolarizing conditions (25 mM KCl) for 24 h at 37 °C and 5% CO 2 in Neurobasal medium (Invitrogen) supplemented with B27 (1:50, Invitrogen), 0.5 mM L -glutamine (Invitrogen) and 25 μg ml −1 gentamycin (Sigma). The slices were also treated either with100 μM TMPyP4, 100 μM TMPyP2 or no drug. All slices were imaged with a Nikon Eclipse 80i fluorescence microscope at 0 and 24 h. How to cite this article: Banerjee, K. et al. Regulation of tyrosine hydroxylase transcription by hnRNP K and DNA secondary structure. Nat. Commun. 5:5769 doi: 10.1038/ncomms6769 (2014).